Photocatalytic hydrogen peroxide splitting on metal-free powders assisted by phosphoric acid as a stabilizer Hydrogen peroxide (H 2 O 2 ) has received increasing attention as an energy carrier. To achieve a sustainable energy society, photocatalytic H 2 O 2 splitting (H 2 O 2 (l) → H 2 (g) + O 2 (g); Δ G ° = + 131 kJ mol −1 ) is a desirable reaction for on-site H 2 generation. However, this reaction has not been reported because conventional photocatalysis decomposes H 2 O 2 by disproportionation (H 2 O 2 (l) → H 2 O (l) + 1/2O 2 (g); Δ G ° = −117 kJ mol −1 ) and by promoting H 2 O 2 reduction instead of H + reduction. Here we report the successful example of H 2 O 2 splitting. Visible light irradiation of a graphitic carbon nitride loaded with graphene quantum dots as co-catalysts (GQDs/g-C 3 N 4 ) in a H 2 O 2 solution containing phosphoric acid (H 3 PO 4 ) produces H 2 . H 3 PO 4 associates with H 2 O 2 via hydrogen bonding, and this stabilization of H 2 O 2 suppresses its reduction, thus promoting H + reduction. The all-organic photosystem with H 3 PO 4 as a stabilizer may provide a basis of photocatalytic H 2 O 2 splitting. Artificial photosynthesis, which transforms earth-abundant resources into fuels by sunlight, is an urgent and challenging issue for realizing a sustainable energy society [1] , [2] . In the last 50 years, photocatalytic water splitting for hydrogen (H 2 ) generation under sunlight irradiation (Eq. ( 1 )) has been extensively studied for this purpose [3] , [4] , [5] . However, H 2 gas has a low volumetric energy density and needs to be converted into a storable and transportable liquid energy carrier such as an organic hydride [6] and ammonia [7] . Therefore, identifying a new artificial photosynthesis system that directly generates a liquid energy carrier is a challenge. Recently, hydrogen peroxide (H 2 O 2 ) has received increasing attention as a new liquid energy carrier because it is storable and transportable and generates electricity in a direct peroxide–peroxide fuel cell (DPPFC), although careful handling is necessary owing to its property of being decomposed in the presence of some metal impurities or under heating conditions [8] . The most attractive feature is that H 2 O 2 can be generated from earth-abundant water and oxygen (O 2 ) via photocatalysis [9] , [10] , [11] . The photogenerated valence band holes (VB h + ) oxidize water (O 2 generation) and the conduction band electrons (CB e − ) reduce O 2 (H 2 O 2 generation). These reactions generate H 2 O 2 by sunlight irradiation under ambient conditions with a positive Gibbs free energy change (Eq. ( 2 )). Therefore, photocatalytic H 2 O 2 generation is a new potential candidate for artificial photosynthesis. Recently, we reported that the resorcinol–formaldehyde resins prepared by the high-temperature hydrothermal synthesis could successfully catalyze the above-mentioned reactions on absorbing visible light up to 620 nm [12] . Further, these metal-free resins stably produced H 2 O 2 with 0.5% of solar-to-chemical conversion efficiency, which is comparable to the highest efficiency for photocatalytic water splitting (Eq. ( 1 )) by metal-based powder photocatalysts [13] . Therefore, H 2 O 2 is a new promising liquid energy carrier candidate. H_2O( l)⟶^hvH_2( g) + 1/2O_2( g)( Δ G^∘ = + 237 kJ mol^-1)
 (1) 
    H_2O( l) + 1/2O_2( g)⟶^hvH_2O_2( l)( Δ G^∘ = + 117 kJ mol^-1)
 (2) To realize a sustainable energy society with H 2 O 2 , on-site generation of H 2 from H 2 O 2 solution is necessary also for its use as a hydrogen carrier. Theoretically, semiconductor photocatalysis can promote the overall H 2 O 2 splitting. The photogenerated VB h + oxidize H 2 O 2 to produce O 2 (Eq. ( 3 )), and the CB e − reduce H + to form H 2 (Eq. ( 4 )). These redox reactions lead to the generation of H 2 from H 2 O 2 under sunlight at ambient temperature (Eq. ( 5 )). Owing to the relatively large Gibbs free energy gain (Δ G ° = +131 kJ mol −1 ), H 2 O 2 splitting is potentially a new type of artificial photosynthesis reaction. Despite these advantages, photocatalytic H 2 O 2 splitting is not reported. This is because H 2 O 2 readily decomposes into water and O 2 over conventional H 2 generation photocatalysts even under dark conditions by disproportionation (Eq. ( 6 )) on the surfaces of metal-oxide semiconductors (such as TiO 2 ) or of metal particle co-catalysts (such as Pt) [14] , [15] , [16] . Other reasons are that H 2 O 2 is decomposed into hydroxyl radicals on ultraviolet (UV) light absorption at λ < 400 nm (Eq. ( 7 )) [17] , [18] , and CB e − reduce H 2 O 2 (Eqs. ( 8 ) and ( 9 )) more efficiently than H + (Eq. ( 4 )), owing to their low-lying reduction potentials [19] . The design of visible-light-driven metal-free photocatalytic systems that can selectively reduce H + while suppressing H 2 O 2 reduction is necessary. H_2O_2( l) + 2h^ + →O_2( g) + 2H^ + ( aq)(  + 0.68V vs NHE)
 (3) 
    2H^ + ( aq) + 2e^- →H_2( g)( 0V vs NHE)
 (4) 
    H_2O_2( l)⟶^hvH_2( g) + O_2( g)( Δ G^∘ = + 131 kJ mol^-1)
 (5) 
    H_2O_2( l) →H_2O( l) + 1/2O_2( g)( Δ G^∘ = -117 kJ mol^-1)
 (6) 
    H_2O_2( l)⟶^hv( λ < 400 nm)2·OH( aq)
 (7) 
    H_2O_2( l) + H^ + ( aq) +  e^- →H_2O( l) + ·OH( aq)(  + 1.14 V vs NHE)
 (8) 
    H_2O_2( l) + 2H^ + ( aq) + 2e^- →H_2O( l)(  + 1.76 V vs NHE)
 (9) Herein, we report the successful example of photocatalytic H 2 O 2 splitting. To avoid the undesirable H 2 O 2 disproportionation (Eq. ( 6 )), we used a graphitic carbon nitride (g-C 3 N 4 ) organic semiconductor [20] . The g-C 3 N 4 is less active for H 2 O 2 disproportionation [14] , and its VB and CB levels (+2.00 and −0.63 V (vs NHE), respectively) are sufficient for H 2 O 2 oxidation (Eq. ( 3 )) and H + reduction (Eq. ( 4 )). We also used graphene quantum dots (GQDs) as co-catalysts; these are the carbon materials belonging to the graphene family and have attracted increasing attention as non-metal H 2 evolution co-catalysts owing to their high electron conductivity and electron reservation capacity [21] , [22] , [23] , [24] . Visible-light irradiation of the GQD/g-C 3 N 4 catalyst in a H 2 O 2 solution containing phosphoric acid (H 3 PO 4 ) at a relatively low temperature (~293 K) successfully produced H 2 . The addition of H 3 PO 4 , which is used as a stabilizer for commercially available H 2 O 2 solution [25] , [26] , plays a pivotal role in this reaction. Raman spectroscopy and ab initio calculations revealed that H 3 PO 4 associates with H 2 O 2 via hydrogen bonding. The stabilization of H 2 O 2 by H 3 PO 4 inhibited H 2 O 2 reduction (Eqs. ( 8 ) and ( 9 )) and, hence, promoted H + reduction (Eq. ( 4 )), resulting in successful H 2 generation. Preparation and characterization of catalyst g-C 3 N 4 powder was prepared by calcination of melamine [27] . The GQDs solution was produced by the reduction of nitrated pyrene with hydrazine followed by hydrothermal treatment [23] . The GQD x /g-C 3 N 4 catalyst was prepared by the hydrothermal treatment of a GQDs solution containing g-C 3 N 4 , where x denotes the amount of GQDs-loaded relative to that of g-C 3 N 4 [ x (wt%) = GQDs/g-C 3 N 4 × 100]. In the UV–visible absorption spectra of the solution (Supplementary Fig. 1 ), the absorption band at λ > 500 nm for GQDs [28] almost disappears completely after hydrothermal treatment with g-C 3 N 4 , indicating that almost all of the GQDs in the solutions were successfully loaded on the g-C 3 N 4 surface. In Fig. 1a , the diffuse-reflectance (DR) UV–visible spectrum of GQD x /g-C 3 N 4 presents a band at λ < 470 nm, which is assigned to the bandgap transition of g-C 3 N 4 . Increasing the amount of the GQDs loaded increases the absorbance at λ > 500 nm, indicating that the GQDs are indeed loaded on the g-C 3 N 4 surface. The bandgap energies of both g-C 3 N 4 and GQD 1 /g-C 3 N 4 were determined to be ~2.6 eV by the Tauc plot analysis (Supplementary Fig. 2 ), suggesting that the GQDs loading scarcely affects the band structure of g-C 3 N 4 . The powder X-ray diffraction (XRD) patterns of g-C 3 N 4 and GQD x /g-C 3 N 4 present peaks at 2 θ = 27.4° ( d = 0.325 nm), which are assigned to the (002) packing of the melem sheet (Supplementary Fig. 3 ) [20] , indicating that these catalysts maintain their layered stacking structure even after the GQDs loading. The scanning electron microscopy (SEM) images of both g-C 3 N 4 and GQD 1 /g-C 3 N 4 (Supplementary Fig. 4 ) indicate an amorphous solid morphology with similar sizes (~30 μm diameter). The transmission electron microscopy (TEM) results of the GQDs solution (Fig. 2 , top) present dispersed GQD particles with ~3-nm diameters [23] , [29] , [30] . In contrast, the GQD 1 /g-C 3 N 4 catalyst (Fig. 2 , bottom) has larger GQD particles with ~10-nm diameters, indicating that the GQD particles are loaded onto the g-C 3 N 4 surface via some aggregation during the hydrothermal treatment. Fig. 1: Properties of GQD x /g-C 3 N 4 photocatalysts. a DR UV-vis spectra of catalysts. b Amounts of H 2 evolved on the respective catalysts in water containing TEOA as a sacrificial electron donor performed in a closed system (0.1 MPa Ar). Conditions: catalyst (100 mg), a water/TEOA (9/1 v/v) mixture (30 mL), light irradiation ( λ > 420 nm, Xe lamp), room temperature, and photoirradiation time (6 h). Error bars represent standard error (s.e.) determined by three independent experiments. c Photocurrent response of the catalysts measured on an FTO glass in 0.1 M Na 2 SO 4 solution at a bias of 0.8 V vs Ag/AgCl. d Time-dependent change in the amount of H 2 evolved and the H 2 selectivity during photoirradiation of the entire wavelength light ( λ > 300 nm) or λ > 420 nm light in a closed gas circulation system (3 kPa Ar). Conditions: catalyst (200 mg), H 2 O 2 (10 mM, 100 mL), H 3 PO 4 (1 M), temperature (293 K), and light irradiation (solar simulator with AM 1.5 G filter, 1-sun). Error bars represent standard error (s.e.) determined by three independent experiments. Full size image Fig. 2: Typical TEM images. a GQD solution. b GQD 1 /g-C 3 N 4 catalyst. The red arrows are the guide for the eyes to follow the GQD particles. Full size image Effect of GQDs as co-catalysts The effect of the GQDs on the photocatalytic activity for H 2 generation was studied using triethanolamine (TEOA) as a sacrificial electron donor. A TEOA/water (1/9 v/v) mixture (30 mL) containing the catalyst (100 mg) was photoirradiated for 6 h by a xenon lamp ( λ > 420 nm) with magnetic stirring at room temperature under Ar atmosphere in a closed system (0.1 MPa). 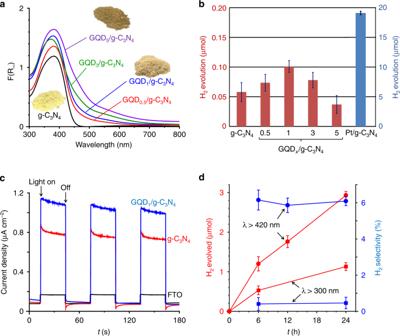Fig. 1: Properties of GQDx/g-C3N4photocatalysts. aDR UV-vis spectra of catalysts.bAmounts of H2evolved on the respective catalysts in water containing TEOA as a sacrificial electron donor performed in a closed system (0.1 MPa Ar). Conditions: catalyst (100 mg), a water/TEOA (9/1 v/v) mixture (30 mL), light irradiation (λ> 420 nm, Xe lamp), room temperature, and photoirradiation time (6 h). Error bars represent standard error (s.e.) determined by three independent experiments.cPhotocurrent response of the catalysts measured on an FTO glass in 0.1 M Na2SO4solution at a bias of 0.8 V vs Ag/AgCl.dTime-dependent change in the amount of H2evolved and the H2selectivity during photoirradiation of the entire wavelength light (λ> 300 nm) orλ> 420 nm light in a closed gas circulation system (3 kPa Ar). Conditions: catalyst (200 mg), H2O2(10 mM, 100 mL), H3PO4(1 M), temperature (293 K), and light irradiation (solar simulator with AM 1.5 G filter, 1-sun). Error bars represent standard error (s.e.) determined by three independent experiments. Figure 1b presents the amount of H 2 evolved over the respective catalysts. The loading of GQDs enhances H 2 evolution, indicating that the GQDs act as co-catalysts for H + reduction. GQD 1 /g-C 3 N 4 exhibits the highest activity; however, further GQDs loading decrease the activity. This decrease is because a larger amount of GQDs absorb more incident light (Fig. 1a ) and suppresses the photoexcitation of g-C 3 N 4 . Figure 1c shows the photocurrent responses of the catalysts measured on a fluorine tin oxide (FTO) electrode. The photocurrent density of GQD 1 /g-C 3 N 4 is higher than that of g-C 3 N 4 , indicating that the CB e − photogenerated on g-C 3 N 4 are efficiently transferred to the GQDs and electrode [31] , [32] . The enhanced charge separation of the h + and e − pairs by the GQDs loading, therefore, enhances the activity for H 2 evolution. As shown by the blue bar in Fig. 1b , g-C 3 N 4 when loaded with Pt particles (Pt/g-C 3 N 4 ), a typical noble metal co-catalyst for H 2 generation [33] , exhibits a much higher activity than GQD 1 /g-C 3 N 4 , where the amount of H 2 formed is 100-fold higher than that formed on GQD 1 /g-C 3 N 4 . The activity of the GQDs as co-catalysts for H 2 generation is lower than that of Pt. Photocatalytic H 2 O 2 splitting Photocatalytic H 2 O 2 splitting was performed in a closed gas circulation system at a reduced pressure [34] (3 kPa Ar) under a constant temperature. Visible light ( λ > 420 nm) was irradiated by a solar simulator with an AM1.5 G filter (1-sun) to a H 2 O 2 solution (1 mmol, 100 mL) containing a catalyst (200 mg) at 293 K. Table 1 lists the amounts of H 2 and O 2 generated and the amount of H 2 O 2 consumed during 6 h of photoirradiation. As shown by entry 1, stirring the solution containing GQD 1 /g-C 3 N 4 in the dark does not produce H 2 or O 2 and does not consume H 2 O 2 , indicating that the catalyst is indeed inactive for the disproportionation of H 2 O 2 . As shown by entry 2, photoirradiation of Pt/g-C 3 N 4 does not produce H 2 while decomposing almost the entire H 2 O 2 and producing a very large amount of O 2 , suggesting that Pt significantly promote H 2 O 2 disproportionation (Eq. ( 6 )) [14] , [15] . As shown by entry 3, photoirradiation of GQD 1 /g-C 3 N 4 in pure water without H 2 O 2 does not produce H 2 or O 2 because g-C 3 N 4 is less active for water oxidation by the VB h + due to its relatively negative VB level [35] . As exhibited by entry 4, photoirradiation of GQD 1 /g-C 3 N 4 in a H 2 O 2 solution also does not produce H 2 while promoting O 2 production (17 μmol) and H 2 O 2 consumption (30 μmol), suggesting that the CB e − do not reduce H + (Eq. ( 4 )) although the VB h + oxidize H 2 O 2 (Eq. ( 3 )). This is because the CB e − reduce H 2 O 2 (Eqs. ( 8 ) and ( 9 )) more efficiently than H + reduction (Eq. ( 4 )), owing to their low-lying reduction potentials [19] . The H 2 O 2 reduction by CB e − must therefore be suppressed to promote H + reduction. Table 1 Results of photocatalytic H 2 O 2 splitting. Full size table Effect of H 3 PO 4 It is well known that H 3 PO 4 is generally added to commercially available H 2 O 2 solutions as a stabilizer to inhibit the decomposition of H 2 O 2 [36] , [37] . Therefore, we studied the effect of H 3 PO 4 on the photocatalytic H 2 O 2 splitting. As exhibited by entries 5–7, visible-light irradiation of GQD 1 /g-C 3 N 4 in a H 2 O 2 solution containing H 3 PO 4 produces H 2 . This is the first successful example of photocatalytic H 2 O 2 splitting. The photocatalytic activity depends on the amount of H 3 PO 4 added. The addition of 1 M H 3 PO 4 (entry 6) produces the largest amount of H 2 (1.2 μmol), but further addition (entry 7) decreases the activity. Several types of reagents such as H 3 PO 3 [37] , uric acid [38] , Na 2 CO 3 [39] , KHCO 3 [40] , barbituric acid [41] , hippuric acid [42] , urea, and acetanilide [43] have also been reported to serve as stabilizers for H 2 O 2 . However, as shown in Supplementary Table 1 , the photoirradiation of GQD 1 /g-C 3 N 4 in a H 2 O 2 solution containing each of the respective reagents barely produces H 2 , indicating that H 3 PO 4 is specifically effective for photocatalytic H 2 O 2 splitting. The pH of 1 M H 3 PO 4 solution is ~1.0. As presented by entry 8, the photoreaction, when performed in a H 2 O 2 solution with H 2 SO 4 (0.1 M, pH ~1), does not produce H 2 . This indicates that a low pH is not a critical factor for enhanced H 2 generation with H 3 PO 4 . As exhibited by entry 7, addition of more H 3 PO 4 (2 M) decreases the amount of H 2 generated. In this case, the amounts of O 2 generated and H 2 O 2 consumed also decrease because the H + concentration increased by a larger amount of H 3 PO 4 (pH ~0.7) suppresses the H 2 O 2 oxidation by the VB h + (Eq. ( 3 )). These data imply that H 3 PO 4 may interact with H 2 O 2 and inhibit its reduction (Eqs. ( 8 ) and ( 9 )), resulting in the promotion of H + reduction (Eq. ( 4 )). As shown by entry 9, the Pt/g-C 3 N 4 catalyst, when photoirradiated with 1 M H 3 PO 4 , produces H 2 ; however, in the absence of H 3 PO 4 , H 2 is not produced (entry 2). This confirms that H 3 PO 4 interacts with H 2 O 2 and inhibits the H 2 O 2 reduction by the CB e − ; however, the amount of H 2 formed (0.2 μmol) is much smaller than that formed over GQD 1 /g-C 3 N 4 (1.2 μmol, entry 6). In this case, almost the entire H 2 O 2 (1 mmol) is decomposed, similar to the case without H 3 PO 4 (entry 2), indicating that Pt particles inevitably promote H 2 O 2 disproportionation even in the presence of H 3 PO 4 (Eq. ( 6 )). Therefore, the use of the all-organic GQD/g-C 3 N 4 catalyst, which is inactive for H 2 O 2 disproportionation, together with H 3 PO 4 , which suppresses H 2 O 2 reduction by the CB e − , is effective for photocatalytic H 2 O 2 splitting. Stabilization of H 2 O 2 by H 3 PO 4 H 3 PO 4 is used as a stabilizer to suppress the disproportionation of H 2 O 2 caused by metal cation impurities [44] , [45] , although the mechanism for their association has not been clarified yet [46] , [47] , [48] . The interaction between H 2 O 2 and H 3 PO 4 was confirmed by cyclic voltammetry (CV) measurements. Figure 3 presents the CV curves obtained with a GQDs-loaded glassy carbon electrode in a solution containing 0.1 M Na 2 SO 4 as an electrolyte. 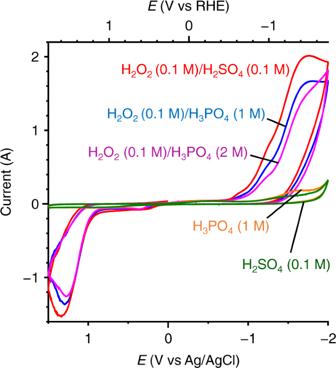Fig. 3: CV charts measured on a GQDs-loaded grassy carbon electrode in the different solutions. The pH of the solutions is ~1, and all the measurements were carried out under N2atmosphere with 0.1 M Na2SO4and at a scan rate of 0.1 V s−1. In 0.1 M H 2 SO 4 (pH ~1.0), as denoted by a green line, the CV curve presents a weak cathodic current at ~ –1.5 V (vs RHE), which is assigned to H + reduction, where no anodic current is observed. The H 3 PO 4 solution (1 M, pH ~1.0) presents a similar CV curve (yellow line). Addition of H 2 O 2 (0.1 M) to the H 2 SO 4 solution (red line) exhibits a strong cathodic current at <–0.8 V, which is assigned to H 2 O 2 reduction (Eqs. ( 8 ) and ( 9 )) [49] , whereas a strong anodic current is observed at >1.2 V, which is assigned to H 2 O 2 oxidation (Eq. ( 3 )). In contrast, as shown by the blue and purple lines, addition of H 2 O 2 to the H 3 PO 4 solution presents cathodic current, which is weaker than that obtained in the H 2 O 2 /H 2 SO 4 mixture (red line). These data indicate that H 2 O 2 interacts with H 3 PO 4 and suppresses its reduction. As reported [50] , at this pH (~1), phosphoric acid exists as a non-dissociated neutral H 3 PO 4 form, where its mole ratio is ~94% and a mole ratio of mono-deprotonated H 2 PO 4 − form is ~6%, suggesting that H 2 O 2 interacts with the H 3 PO 4 form. Fig. 3: CV charts measured on a GQDs-loaded grassy carbon electrode in the different solutions. The pH of the solutions is ~1, and all the measurements were carried out under N 2 atmosphere with 0.1 M Na 2 SO 4 and at a scan rate of 0.1 V s −1 . Full size image Raman spectroscopy The interaction between H 2 O 2 and H 3 PO 4 was further studied via Raman spectroscopy at 293 K (Fig. 4a ). Pure water (purple) exhibits a strong band at 2800–3800 cm −1 for the O–H stretching vibration of water, indicative of strong hydrogen (H-) bonding between the water molecules, as is schematically shown in Fig. 5a (left). The H 2 O 2 solution (black) exhibits a weaker O–H band because the interaction between H 2 O 2 and water weakens the H-bonding between the water molecules. The H 3 PO 4 solution (orange) exhibits a much weaker O–H band because, as shown in Fig. 5a (middle), H 3 PO 4 strongly interacts with water [50] and significantly weakens the H-bonding between the water molecules. The addition of H 2 O 2 to the H 3 PO 4 solution (blue), however, increases the O–H band. This indicates that, as shown in Fig. 5a (right), H 3 PO 4 interacts with H 2 O 2 more strongly than with water owing to the H-bonding interaction to form the H 2 O 2 –H 2 PO 4 − bidentate complex with a structure similar to the urea–H 2 PO 4 − complex [51] . This may suppress the water–H 3 PO 4 interaction and regenerate strong H-bonding interaction between the water molecules. These data suggest that H 3 PO 4 associates with H 2 O 2 via H-bonding to form a stabilized complex (Fig. 5a (right)), which may inhibit the H 2 O 2 reduction by the CB e − . 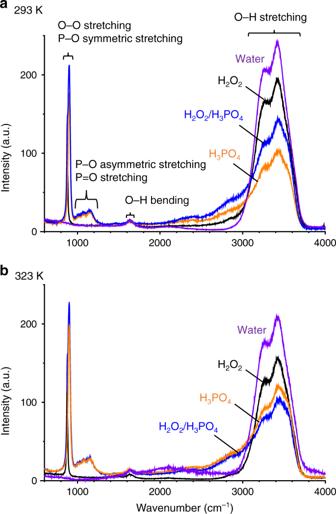Fig. 4: Raman spectra (600–4000 cm−1region) of the respective solutions. a293 K.b323 K. The H2O2and H3PO4concentrations are 2 M and 4 M, respectively. Fig. 4: Raman spectra (600–4000 cm −1 region) of the respective solutions. a 293 K. b 323 K. The H 2 O 2 and H 3 PO 4 concentrations are 2 M and 4 M, respectively. Full size image Fig. 5: Schematic representation of H-bonding interaction and optimized structures of compounds. a Sequential change in H-bonding interaction between water, H 2 PO 4 − , and H 2 O 2 . b optimized structures of H 2 O 2 , H 2 PO 4 − , and H 2 O 2 –H 2 PO 4 − complex (DFT/B3LYP/6–31 G*(d), PCM: water). Full size image Figure 6a presents the Raman spectroscopy results of the respective solutions in the 850–950 cm −1 region measured at 293 K. The H 2 O 2 solution (top) exhibits a band at 875.6 cm −1 , which is assigned to the O–O stretching vibration of H 2 O 2 [52] . The H 3 PO 4 solution (middle) exhibits a band at 899.0 cm −1 assigned to the P–O symmetric stretching vibration of H 3 PO 4 [53] . 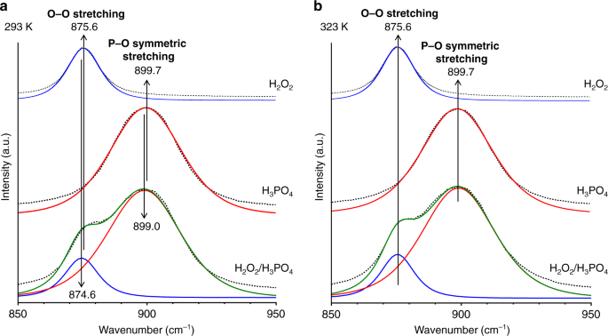Fig. 6: Raman spectra (850–950 cm−1) of (top) H2O2, (middle) H3PO4, and (bottom) a mixture of H2O2and H3PO4measured at different temperatures. a293 K.b323 K. The H2O2and H3PO4concentrations are 2 M and 4 M, respectively. The dots are the experimental data, and the solid lines are the deconvoluted components, where the green lines are the sum of the components. The spectrum of the H 2 O 2 /H 3 PO 4 mixture (bottom) can be deconvoluted into O–O and P–O stretching components. The O–O band of the mixture appears at 874.6 cm −1 , which lies at a lower wavenumber (Δ \(\widetilde v\) = −1.0 cm −1 ) than that of the band of pure H 2 O 2 (875.6 cm −1 ). In addition, the P–O band of the mixture appears at 899.0 cm −1 , which also lies at a lower wavenumber (Δ \(\widetilde v\) = −0.7 cm −1 ) than that of pure H 3 PO 4 (899.7 cm −1 ). These data suggest that the lengths of the O–O and P–O bonds are extended by the H-bonding between H 2 O 2 and H 3 PO 4 (Fig. 5a (right)). Fig. 6: Raman spectra (850–950 cm −1 ) of (top) H 2 O 2 , (middle) H 3 PO 4 , and (bottom) a mixture of H 2 O 2 and H 3 PO 4 measured at different temperatures. a 293 K. b 323 K. The H 2 O 2 and H 3 PO 4 concentrations are 2 M and 4 M, respectively. The dots are the experimental data, and the solid lines are the deconvoluted components, where the green lines are the sum of the components. Full size image Ab initio calculations To obtain further information on the interaction between H 2 O 2 and H 3 PO 4 , the structure of the H 2 O 2 –H 2 PO 4 − complex (Fig. 5a (right)) was calculated by density functional theory (DFT) using the polarizable continuum model (PCM) with water as the solvent (Supplementary Tables 3 – 6 ) [54] . 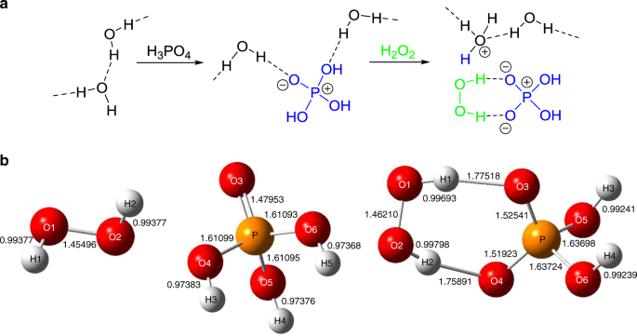Figure 5b presents the optimized structures of H 2 O 2 , H 3 PO 4 , and the H 2 O 2 –H 2 PO 4 − complex, and the lengths of the respective bonds. Fig. 5: Schematic representation of H-bonding interaction and optimized structures of compounds. aSequential change in H-bonding interaction between water, H2PO4−, and H2O2.boptimized structures of H2O2, H2PO4−, and H2O2–H2PO4−complex (DFT/B3LYP/6–31 G*(d), PCM: water). 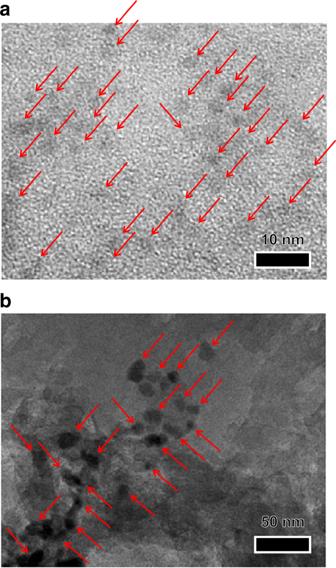The O–O bond length in the complex (1.462 Å) is longer than that in H 2 O 2 (1.455 Å). In addition, the lengths of the two P–O bonds in the complex (1.525 Å (P–O3) and 1.519 Å (P–O4)) are longer than those in H 3 PO 4 (1.480 Å (P–O3)), where the average P–O lengths of the complex (1.580 Å) is also longer than those of H 3 PO 4 (1.578 Å). The shortened lengths of the O–O bond (Δ = 0.007 Å) and P–O bonds (Δ = 0.002 Å) by the H-bonding interaction agree reasonably with the lower wavenumber shift of the O–O and P–O stretching vibrations, as confirmed via Raman analysis (Fig. 6a ). Fig. 2: Typical TEM images. aGQD solution.bGQD1/g-C3N4catalyst. The red arrows are the guide for the eyes to follow the GQD particles. The DFT frequency calculations (Supplementary Table 2 ) reveal that the wavenumbers of the O–O stretching in H 2 O 2 and the complex are 947.7 cm −1 and 942.8 cm −1 [55] , respectively (Δ \(\widetilde v\) = −4.9 cm −1 ), and the wavenumbers of the P–O symmetric stretching in H 3 PO 4 and the complex are 1075 cm −1 and 1039 cm −1 [56] , respectively (Δ \(\widetilde v\) = −36 cm −1 ). Although the frequencies calculated by DFT are overestimated owing to the large anharmonicity of the high-frequency modes [57] , [58] , the lower wavenumber shifts of the O–O and P–O bonds caused by the H-bonding interaction between H 2 O 2 and H 3 PO 4 are consistent with the Raman data (Fig. 6a ). In addition, the two O–H‧‧‧O distances of the complex are 2.749 Å (O1–H1‧‧‧O3) and 2.733 Å (O2–H2‧‧‧O4), indicative of strong and mostly electrostatic H-bonding interaction between H 2 O 2 and H 3 PO 4 [59] . Supplementary Fig. 5 summarizes the energy diagram for the frontier molecular orbitals [60] of the calculated models. The interaction of the highest-occupied molecular orbital (HOMO) of H 2 PO 4 − with the lowest-unoccupied molecular orbital (LUMO) of H 2 O 2 creates a frontier orbital of the complex (LUMO + 1) at an energy level higher than that of free H 2 O 2 , meaning that the H 2 O 2 moiety of the complex is stabilized against its reduction upon external electron injection [61] . This is because the electron donation from H 2 PO 4 − to H 2 O 2 leads to a decrease in the electron affinity of the H 2 O 2 moiety and stabilizes its orbital. The result is consistent with the suppressed H 2 O 2 reduction (Fig. 3 ) and the enhanced H 2 evolution (Table 1 , entry 6) by the addition of H 3 PO 4 . Therefore, H 3 PO 4 associates with H 2 O 2 via H-bonding and produce a stabilized complex (Fig. 5a (right) and Fig. 5b (right)). This interaction decreases the electron affinity of H 2 O 2 and suppresses the H 2 O 2 reduction by the CB e − (Eqs. ( 8 ) and ( 9 )), thus resulting in the promotion of H + reduction (Eq. ( 4 )). It must be noted that addition of H 3 PO 4 is necessary for efficient stabilization of H 2 O 2 ; addition of phosphate salts is ineffective. As shown by entry 10 (Table 1 ), a NaH 2 PO 4 (1 M) solution (pH ~1), when used for photoreaction, produces a lower amount of H 2 than a H 3 PO 4 (1 M) solution (entry 6) although fully protonated H 3 PO 4 species exist in both solutions. Alkaline metal cations interact with H 2 O 2 in solution [62] . The H 2 O 2 –Na + interaction may weaken the H 2 O 2 –H 2 PO 4 − complex, probably resulting in the decreased H 2 evolution activity. Temperature effect The stability of the H 2 O 2 –H 2 PO 4 − complex depends on the temperature of the solution. As shown by entry 6 (Table 1 ), the photoirradiation of GQD 1 /g-C 3 N 4 at 293 K in a H 2 O 2 solution containing 1 M H 3 PO 4 produces 1.2 μmol of H 2 . However, when the reaction is performed at 303 K (entry 11), the amount of H 2 produced is decreased to 0.5 μmol, and further increase in the temperature (313 K and 323 K) does not produce H 2 (entries 12 and 13), indicating that higher temperature is ineffective. To clarify the temperature effect on the H 2 O 2 –H 2 PO 4 − interaction, Raman spectroscopy was measured at a high temperature (323 K). As displayed in Fig. 4b (orange), the O–H band of water decreases by the addition of H 3 PO 4 ; this is owing to the water–H 3 PO 4 H-bonding interaction (Fig. 5a (middle)), similar to the case at 293 K (Fig. 4a ). At 293 K, the decreased O–H band increases on the addition of H 2 O 2 ; this is because the formation of the H 2 O 2 –H 2 PO 4 − complex regenerates the H-bonding between the water molecules. However, at 323 K, the addition of H 2 O 2 to the H 3 PO 4 solution barely increases the O–H band, indicating that there is no H-bonding interaction between H 2 O 2 and H 2 PO 4 − . As displayed in Fig. 6a , the Raman spectrum of the H 2 O 2 /H 3 PO 4 mixture measured at 293 K presents O–O (874.6 cm −1 ) and P–O (899.0 cm −1 ) bands, both of which lie at lower wavenumbers than those of only H 2 O 2 (875.6 cm −1 ) and H 3 PO 4 (899.7 cm −1 ), owing to the H 2 O 2 –H 2 PO 4 − complex formation. However, at 323 K (Fig. 6b ), the H 2 O 2 /H 3 PO 4 mixture shows O–O (875.6 cm −1 ) and P–O (899.7 cm −1 ) bands at identical positions to those in H 2 O 2 and H 3 PO 4 . These data suggest that the H 2 O 2 –H 2 PO 4 − complex is destabilized at higher temperatures because a rise in temperature increases the kinetic energy of the molecules and weakens their H-bonding interaction [63] , as observed in several H-bonding systems such as dimethyl sulfoxide–water [64] and urea–water [65] at the similar temperature range (283–333 K). The weakened interaction at higher temperatures inevitably promotes H 2 O 2 reduction (Eqs. ( 8 ) and ( 9 )) and, hence, decrease H 2 generation (Eq. ( 4 )). The photoreaction at a relatively lower temperature is therefore necessary for efficient H 2 generation. Effect of light wavelength Visible-light irradiation is also necessary for this system. Figure 1d shows the time course for the amount of H 2 evolved during the photocatalytic H 2 O 2 splitting over the GQD 1 /g-C 3 N 4 catalyst with 1 M H 3 PO 4 at 293 K. Further, the H 2 selectivity is defined as the ratio of the amount of H 2 evolved to that of the consumed H 2 O 2 (Eq. ( 10 )). Under visible light ( λ > 420 nm) exposure, as depicted by circle keys, the amount of H 2 evolved increases almost linearly with time, and the H 2 selectivity is almost constant even after prolonged photoirradiation. This indicates that the system consisting of the all-organic GQD 1 /g-C 3 N 4 catalyst and H 3 PO 4 as a stabilizer at a low temperature stably promotes H 2 O 2 splitting. In addition, as presented in Supplementary Fig. 6 , the recovered GQD 1 /g-C 3 N 4 catalyst, when reused for further photoreactions, maintains the activity and the H 2 selectivity, indicating that the catalyst is reusable without the loss of activity. However, the H 2 selectivity is only ~6 %, indicating that the H 2 O 2 reduction (Eqs. ( 8 ) and ( 9 )) still occurs more efficiently than the H + reduction (Eq. ( 4 )) even in the presence of H 3 PO 4 . H_2 selectivity( %) = [ H_2 evolved( mol)]/[ H_2O_2 consumed( mol)]× 100
 (10) The square keys in Fig. 1d denote the results obtained under irradiation of the entire wavelength light ( λ > 300 nm) from the solar simulator (Supplementary Fig. 7 ). The amount of H 2 evolved is much smaller than that under λ > 420 nm irradiation. As summarized in Table 1 (entry 14), λ > 300 nm irradiation for 6 h produces a larger amount of O 2 (22 μmol) than the λ > 420 nm irradiation (7.7 μmol, entry 5). This indicates that UV irradiation enhances the catalyst photoexcitation and efficiently promotes H 2 O 2 oxidation by the VB h + (Eq. ( 3 )), clearly suggesting that UV irradiation suppresses H + reduction (Eq. ( 4 )). The λ > 300 nm irradiation decomposes a larger amount of H 2 O 2 (127 μmol) than the λ > 420 nm irradiation (20 μmol, entry 6); this is owing to the photodecomposition of H 2 O 2 by the absorbed UV light (Eq. ( 7 )), as confirmed by the absorption spectra of the H 2 O 2 solution in the UV region (Supplementary Fig. 8 ). This suggests that the H 2 O 2 –H 2 PO 4 − complex absorbs UV light and undergoes destabilization. The weakened H-bonding of the complex may therefore inevitably promote H 2 O 2 reduction (Eqs. ( 8 ) and ( 9 )), thus inhibiting the H + reduction (Eq. ( 4 )). As displayed in Fig. 1d (square), the H 2 selectivity with λ > 300 nm irradiation is only ~0.5% owing to the accelerated H 2 O 2 decomposition, indicating that visible-light irradiation is necessary for efficient photocatalytic H 2 O 2 splitting. Even under visible-light irradiation, the H 2 selectivity is ~6%; therefore, further selectivity enhancement is necessary for practical applications. Nevertheless, the successful example presented here based on the combination of an all-organic photocatalyst and H 3 PO 4 as a stabilizer under sunlight illumination presents significant potential for photocatalytic H 2 O 2 splitting. Visible-light irradiation of the all-organic GQD/g-C 3 N 4 catalyst in a H 2 O 2 solution containing H 3 PO 4 at a relatively low temperature (~293 K) could successfully promote H 2 generation by photocatalytic H 2 O 2 splitting. The Raman spectroscopy and DFT calculations revealed that H 3 PO 4 associates with H 2 O 2 via H-bonding interaction and forms a H 2 O 2 –H 2 PO 4 − complex at a low temperature. This decreases the electron affinity of H 2 O 2 and suppresses its reduction, thus promoting H + reduction (H 2 generation). The present system stably produces H 2 even after prolonged photoirradiation, and the catalyst is reusable without the loss of activity and H 2 selectivity. This photocatalytic system offers several advantages: a metal-free photocatalyst and inexpensive acid (H 3 PO 4 ) can be used for the reaction; visible light, a main constituent of sunlight irradiation, can be used as the light source; and on-site H 2 generation from a transportable and storable energy carrier (H 2 O 2 ) can be achieved. At present, H 2 selectivity is only ~6% relative to the amount of H 2 O 2 consumed, and further improvement of its selectivity is necessary for practical applications. Nevertheless, the successful example presented here based on an all-organic catalyst with H 3 PO 4 as a stabilizer may contribute to the design of a highly efficient system for the on-site photocatalytic generation of H 2 from a H 2 O 2 solution. Catalyst preparation The g-C 3 N 4 powder was prepared by calcination of melamine at 823 K (heating rate: 2.3 K min −1 , holding time: 4 h) [27] . The GQDs solution was synthesized as follows: [30] pyrene (2 g) was stirred in concentrated HNO 3 (160 mL) at 353 K for 12 h. Water (2 L) was added to the resultant, and the solids formed were recovered by filtration. The solids were dispersed in hydrazine hydrate solution (1.0 M, 40 mL), ultrasonicated for 2 h, and left in an autoclave at 423 K for 10 h. Filtration of the resultant by a microporous membrane afforded a 0.5-g L −1 GQDs solution. The GQD x /g-C 3 N 4 catalysts [ x (wt%) = 0.5, 1.0, 3.0, and 5.0] were prepared as follows: g-C 3 N 4 (0.4 g) was added to 40 mL of the GQDs solution (0.05, 0.1, 0.3, and 0.5 g L −1 ) and stirred for 1 h at 298 K. The mixture was left in an autoclave at 423 K for 4 h. The solids were recovered by centrifugation, washed with water, and dried at 353 K, affording GQD x /g-C 3 N 4 as brown powders. A Pt/g-C 3 N 4 catalyst (Pt loading: 0.3 wt%) was prepared as follows: [33] g-C 3 N 4 (1.0 g) was added to water (30 mL) containing H 2 PtCl 6 ‧6H 2 O (8.0 mg) and evaporated with vigorous stirring at 373 K. The obtained powders were reduced under H 2 flow (0.1 mL min −1 ) at 673 K (heating rate: 10 K min −1 , holding time: 2 h). Photoreaction H 2 generation from a TEOA solution was performed in a closed system (0.1 MPa). The catalyst (100 mg) was added to a 10 vol% TEOA solution (30 mL) within a glass tube (φ 35 mm; capacity, 50 mL). The tube was sealed with a rubber cap and ultrasonicated for 5 min, and Ar gas was bubbled through the solution for 10 min. The tube was photoirradiated ( λ > 420 nm) using a 2-kW Xe lamp (USHIO Inc.) with magnetic stirring at room temperature. After the reaction, the amount of H 2 formed was determined by gas chromatography-thermal conductivity detector (GC-TCD) (Shimadzu; GC-8A). Photocatalytic H 2 O 2 splitting was performed in a closed gas circulation system connected to GC-TCD [66] . The catalyst (200 mg) was added to a H 2 O 2 solution (1 mmol, 100 mL) within a quartz cell. The cell was connected to a gas circulation system, and the system was depressurized to 3 kPa after repeated Ar purging. The cell was immersed in a temperature-controlled water bath (±0.1 K) and photoirradiated at λ > 420 nm using a solar simulator equipped with AM1.5 G filter (SAN-EI Electric Inc.; XES-40S3, 1-sun) with magnetic stirring [12] . The amounts of H 2 O 2 in the solutions were determined by redox titration with KMnO 4 . Analysis The electrochemical measurements were performed in a conventional three-electrode cell using an electrochemical system (ALS700E, BAS Inc.), where Ag/AgCl and Pt wire electrodes were used as the reference and counter electrodes, respectively [66] . For the photocurrent measurements, a catalyst-loaded FTO glass was used as the working electrode. Catalyst (20 mg) was added to a mixture of water (4 mL), 2-propanol (1.5 mL), and 5 wt% Nafion solution (100 μL) [67] , and ultrasonicated for 10 min. The slurry was placed onto an FTO glass and dried at room temperature. The film was formed to 0.5 cm × 0.5 cm square, where the undeposited parts were coated with an epoxy resin. For the CV measurements, a glassy carbon electrode loaded with GQD was used as the working electrode, where the GQD solution was placed on the electrode and dried at room temperature. All the measurements were performed after N 2 bubbling through the solution for 1 h. Raman spectra were measured on a confocal Raman microscope (LabRAM HR-800, HORIBA) with a YAG laser (532 nm line) as the excitation source, where the laser power was 100 mW and the total data accumulation time was 100 s, respectively. DR UV-vis, XRD, SEM, and TEM observations were performed according to the procedures described in the literature [12] . Computational details The molecular structures were optimized by the B3LYP functional (B3LYP/6-31G*(d)) using the polarizable continuum model (PCM) with water as the solvent [54] in the Gaussian 03 program. Cartesian coordinates for the models used are summarized at the end of the Supplementary Material.